Molecular cobalt corrole complex for the heterogeneous electrocatalytic reduction of carbon dioxide Electrochemical conversion of CO 2 to alcohols is one of the most challenging methods of conversion and storage of electrical energy in the form of high-energy fuels. The challenge lies in the catalyst design to enable its real-life implementation. Herein, we demonstrate the synthesis and characterization of a cobalt(III) triphenylphosphine corrole complex, which contains three polyethylene glycol residues attached at the meso -phenyl groups. Electron-donation and therefore reduction of the cobalt from cobalt(III) to cobalt(I) is accompanied by removal of the axial ligand, thus resulting in a square-planar cobalt(I) complex. The cobalt(I) as an electron-rich supernucleophilic d 8 -configurated metal centre, where two electrons occupy and fill up the antibonding d z 2 orbital. This orbital possesses high affinity towards electrophiles, allowing for such electronically configurated metals reactions with carbon dioxide. Herein, we report the potential dependent heterogeneous electroreduction of CO 2 to ethanol or methanol of an immobilized cobalt A 3 -corrole catalyst system. In moderately acidic aqueous medium (pH = 6.0), the cobalt corrole modified carbon paper electrode exhibits a Faradaic Efficiency (FE%) of 48 % towards ethanol production. Minimizing of the CO 2 concentration in the atmosphere is one of the most important challenges in our time [1] , [2] . Therefore, the electrochemical reduction of CO 2 to value added chemicals is a sustainable strategy to solve the growing energy crisis, which at the same time has the potential to mitigate environmental pollution. In the past years, the electrochemical reduction of CO 2 has been studied by several research groups to produce valuable products, for example carbon monoxide, formic acid, methane, ethanol, or methanol [3] , [4] , [5] . Particularly the transformation of CO 2 in high-density alcohols, especially methanol and ethanol, is a cherished goal for chemists and environmental engineers alike [6] , [7] . Such transformation of CO 2 to alcohols coupled with the oxidation of water to oxygen [8] is a promising strategy [9] . However, the low reactivity of carbon dioxide in water with its large energy barrier (∆ E = −1366.8 kJ mol −1 ) [10] and the competing hydrogen evolution reaction, impedes such transformation, which makes the development of catalysts for electrocatalytic CO 2 reduction to ethanol in aqueous environment a big challenge [1] , [2] , [10] . The thermodynamic reduction potential for CO 2 to methanol and ethanol is 0.03 and 0.09 V (vs. RHE), respectively which is kinetically disfavored. Hence, often CO 2 reducing catalysts end up accruing lot of energy to be operational at a higher potential. In this regard the use of a molecular catalyst with earth abundant elements, (Fe, Mn, Co, Cu, and Ni), especially with a cobalt metal center [11] , [12] is a viable alternative as it offers a high degree of tunability with product selectivity at a low overpotential. As early as in 1980s chemists have been successful in reducing CO 2 to CO via electrochemical methods employing catalysts containing different metals like Co [13] , Ni [14] , Re [15] , [16] , [17] , etc. Recently electrochemical reduction of CO 2 to ethanol has been studied in various ways [18] , [19] , by tuning the applied potential [20] , pH [21] , and nature of the electrolyte [22] with an aim to control the product selectivity and increase the Faradaic efficiency (FE) as well as to understand the underlying mechanistic pathways. Metal surfaces [23] , [24] , oxides [25] , and alloys [26] , [27] are the most explored examples which show good FE for CO 2 reduction but lack selectivity [28] , [29] and work at higher overpotentials, involving complex synthetic procedures [30] , [31] . Emergent materials like B and N co-doped nanodiamonds exhibit excellent FE (93 %) and selectivity for conversion to ethanol, but work at higher overpotentials [10] . Moreover such heteroatom-doped materials [32] often require a sophisticated synthetic procedure like chemical vapor deposition, making it hard for large scale implementation [33] . 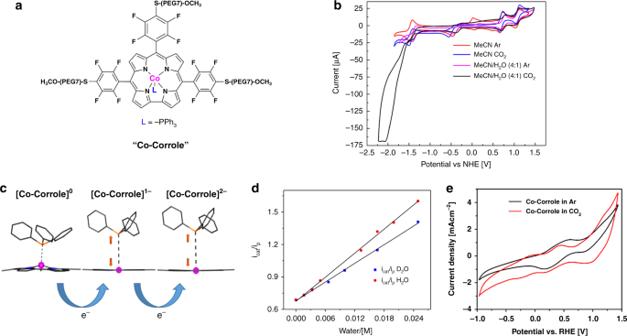Fig. 1 aChemical structure of the Co-corrole.bCyclic voltammetry of Co-corrole dissolved in CH3CN under Ar (red). Two metal centered redox peaks at −0.5 V (Co (III)/Co(II)) and −1.5 V (Co(II)/Co(I)) vs. NHE could be identified. The irreversibility of the redox peak at −0.5 V is likely due to the partial loss of the PPh3ligand. Cyclic voltammetry of Co-corrole dissolved in CH3CN under CO2(blue), in CH3CN/H2O (4:1) under Ar (pink) and in CH3CN/H2O (4:1) under CO2(black).cDFT optimized geometries of [Co-corrole]0, 1e−and 2e−reduced species showing the movement of Co center into the central cavity of the corrole ring with concomitant lengthening of the Co-PPh3bond upon successive reduction.dKinetic isotpopic effect demonstrated by cyclic voltammetry of Co-Corrole (0.5 mM) recorded in CO2saturated in acetonitrile in the presence of varying amount of H2O or D2O. Linear dependence oficat/ipon the concentration of water (analogous to plotting √kCO2vs. [water], KIE = kCO2H/kCO2D= (SlopeH2O/slopeD2O)2= (37.1057/28.7545)2= 1.67). All cyclic voltammograms were recorded with 0.1 M TBAPF6as supporting electrolyte using a glassy carbon as working electrode and a Ag/AgCl as reference electrode at a scan rate of 100 mV s−1.eHeterogeneous catalysis of 1 mM Co-corrole on carbon-fiber electrode under Ar (black) and CO2(red) at pH = 6.0 (Ag/AgCl/KCl, Pt, 0.1 M NaClO4, 100 mV s−1) We now compare and contrast state of the art catalysts for CO 2 electro-reduction to ethanol, all of which work at higher overpotentials with shorter activity time and have lower FE as compared to the catalyst reported here (Supplementary Table 1 ). For instance, Cu(100) works at −0.97 V vs. RHE yielding ethanol with a FE% of 14.7 [29] . Further, use of Cu based nano-particles in an ensemble fashion (trans-CuEn) showed a FE% of ethanol formation to be 17 at −0.86 V vs. RHE [34] . While, with tailoring of cubic Cu nanocrystals to an edge length of 44 nm, FE% of 80 was achieved for CO 2 reduction but the FE% for Ethanol formation was as low as 3.7 [35] . On the other hand, alloys like Cu x Zn show that both the selectivity and FE% of ethanol formation can be governed by tuning the Cu:Zn ratio in the catalyst with a maximum FE% of ethanol formation 29.1 and current density (−3.8 mA cm −2 ) obtained for Cu 4 Zn at −1.05 V vs. RHE [36] . Similarly, electrodeposited Cu–Ag alloy films (6% Ag) exhibit a FE% of ethanol formation to be 25 at −0.7 V vs. RHE with a relatively high current density of −300 mA cm −2 [37] . Ethanol was also obtained by tuning the layer thickness of Cu(I)oxide catalysts with a FE% of 9–16 (current density −35 mA cm −2 ) at −0.99 V vs. RHE [38] , while Cu 2 O derived Cu films exhibit FE% of 11.8 at −0.88 V vs. RHE with a current density of −31.2 mA cm −2 [39] . Materials like nanodiamonds on B and N co-doping shows a very good FE% of 93 and selectivity toward ethanol [10] . With the aim to synthesize effective and stable electrocatalysts for CO 2 reduction for the selective ethanol formation, we focus on a molecular Co-corrole catalyst. Metal corroles are structural similar to metal porphyrins with both the metal centers and ligands participating in multielectron redox processes and are promising candidates for efficient proton-coupled electron transfer [40] , [41] , [42] . These metal complexes stabilize radical intermediates thus providing an effective pathway to facilitate C–C step-up [43] , [44] . Cobalt and iron corroles have been previously found to be catalytically active for CO 2 reduction to CO [12] . We thus explore this class of catalysts for CO 2 electroreduction by using cobalt triphenylphosphine 5,10,15-tris(2,3,5,6-tetrafluoro-4-(MeO-PEG(7))thiophenyl) corrole Co(PPh 3 ) (TpFPC) (-S-PEG(7)-OMe) 3 (“Co-corrole”) where all the three pentafluorophenyl-groups on the meso- positions 5, 10, 15 are modified at the para- positions by thiol bound PEG(7)-OMe moieties [45] , [46] , [47] . In the present work, we demonstrate the reduction of CO 2 to alcohols, formaldehyde, carboxylates, and hydrogen with a Co-corrole modified carbon paper electrode working at a low overpotential (−0.8 V vs. RHE) and show the long-term activity of Co-corrole modified carbon paper electrodes, making it as robust as metallic copper electrocatalysts. The molecular cobalt(III)-corrole catalyst is a significant improvement in the matter of selective reduction of CO 2 to value added chemicals. Synthesis and electrochemical characterization of the catalyst The Co-corrole was synthesized via four steps, where the first two steps leading to 5,10,15-trispentafluorophenylcorrole, were performed according to Gryko’s procedure [48] . The electron-withdrawing properties of the C 6 F 5 functionalities render the corrole ring electron deficient [49] . Chemical modification with the -S-PEG(7)-OMe moieties at the three para- positions of the meso -C 6 F 5 groups was performed (Fig. 1a ) to optimize anchoring and equal distribution of the catalyst on the electrode surface. The chemical syntheses and characterizations are described in detail in the methods section and in the Supplementary Information file (Supplementary Figs. 1 – 6 ). The immobilization process of Co-corrole over carbon paper is implemented via drop casting by using anacetonitrile solution of Co-corrole. The modified carbon paper electrodes are stable in aqueous solution due to the insolubility of the Co-corrole moiety in water resulting in the formation of a sustainable heterogenized catalyst with extended life-time for electrocatalysis. Fig. 1 a Chemical structure of the Co-corrole. b Cyclic voltammetry of Co-corrole dissolved in CH 3 CN under Ar (red). Two metal centered redox peaks at −0.5 V (Co (III)/Co(II)) and −1.5 V (Co(II)/Co(I)) vs. NHE could be identified. The irreversibility of the redox peak at −0.5 V is likely due to the partial loss of the PPh 3 ligand. Cyclic voltammetry of Co-corrole dissolved in CH 3 CN under CO 2 (blue), in CH 3 CN/H 2 O (4:1) under Ar (pink) and in CH 3 CN/H 2 O (4:1) under CO 2 (black). c DFT optimized geometries of [Co-corrole] 0 , 1e − and 2e − reduced species showing the movement of Co center into the central cavity of the corrole ring with concomitant lengthening of the Co-PPh 3 bond upon successive reduction. d Kinetic isotpopic effect demonstrated by cyclic voltammetry of Co-Corrole (0.5 mM) recorded in CO 2 saturated in acetonitrile in the presence of varying amount of H 2 O or D 2 O. Linear dependence of i cat / i p on the concentration of water (analogous to plotting √k CO2 vs. [water], KIE = k CO2H /k CO2D = (Slope H2O /slope D2O ) 2 = (37.1057/28.7545) 2 = 1.67). All cyclic voltammograms were recorded with 0.1 M TBAPF 6 as supporting electrolyte using a glassy carbon as working electrode and a Ag/AgCl as reference electrode at a scan rate of 100 mV s −1 . e Heterogeneous catalysis of 1 mM Co-corrole on carbon-fiber electrode under Ar (black) and CO 2 (red) at pH = 6.0 (Ag/AgCl/KCl, Pt, 0.1 M NaClO 4 , 100 mV s −1 ) Full size image Electrochemical properties of the Co-corrole were investigated by cyclic voltammetry, with glassy carbon as working electrode in CH 3 CN under Argon and 0.1 M TBAPF 6 as supporting electrolyte. As shown in Fig. 1b , red curve, two one electron redox peaks at −0.5 V (Co(III)/Co(II)) and −1.5 V (Co(II)/Co(I)) vs. NHE are occurring (Supplementary Fig. 7 ). The irreversibility of the redox peak at −0.5 V is likely due to the partial loss of the PPh 3 ligand [50] . In analogy to previous report by Kadish et al. [50] , these two couples Co(III)/Co(II) and Co(II)/Co(I) are metal centered redox processes. The reversible two one electron redox peaks at 0.73 and 1.12 V vs. NHE are ligand centered oxidations and correspond to the formation of a cationic and dicationic cobalt(III) corrole complex [50] . DFT calculations suggest that the one-step and the two-step reduction at −0.5 and −1.5 V of the cobalt(III)-corrole leads to enhanced π-back bonding which strengthens the Co–N bonds and the cobalt corrole macrocycle becomes planar (Fig. 1c ). Therefore, demetallation is energetically disfavored, which enables catalysis at a single Co(I)-site. The cyclic voltammetry of Co-corrole under CO 2 (Fig. 1b , black curve) dissolved in CH 3 CN/H 2 O (4:1) shows compared with Co-corrole in ACN under CO 2 (Fig. 1b , blue curve) a steep increase in current at −1.5 V vs. NHE, which confirms that CO 2 reduction occurs in presence of a proton source. A value for the kinetic isotopic effect KIE = 1.64 was determined from the linear plots of i cat / i p against [H 2 O] or [D 2 O] measured at 100 mV s −1 (Fig. 1d ). Cyclic voltammetry of the Co-corrole modified carbon–fiber electrode under Ar (Fig. 1e , black curve) and CO 2 (Fig. 1e , red curve) was investigated in aqueous conditions at pH = 6.0, 7.2, and 8.0 (Supplementary Figs. 8 – 14 , Co-corrole physisorbed on carbon paper). In all cases, a steep increase in catalytic current could be detected at a potential of −0.8 to −1.0 V vs. RHE where the second reduction reaction of [Co-corrole] − to [Co-corrole] 2− occurs (Fig. 1e ). Characterization of the electrocatalyst on the electrode surface Cobalt triphenylphosphine 5,10,15–tris(2,3,5,6-tetrafluoro-4-(MeO-PEG(7))thiophenyl) corrole, Co(PPh 3 ) (TpFPC) (-S-PEG(7)-OMe) 3 (“Co-corrole”), is deposited on carbon paper (fabricated via drop casting using a acetonitrile mixture). 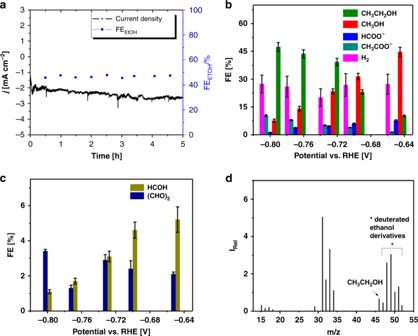Fig. 2 aConstant potential electrolysis of electrochemical CO2reduction by the Co-corrole modified carbon paper electrode at a potential of −0.8 V vs. RHE (black curve), Faradaic efficiency for ethanol production over 5 h electrolysis (blue rectangles).bFE% vs. potential plot for potential dependent product formation.cFE% vs. potential plot for minor formed formaldehyde and solvated dimer of formaldehyde at different potentials. The error bars represent standard deviation of six measurements (three electrochemical reactions with two product analysis measurements for each reaction).dMS spectra obtained after electrolysis at −0.8 V vs. RHE in (1:3) D2O/H2O 0.1 M NaClO4saturated with CO2 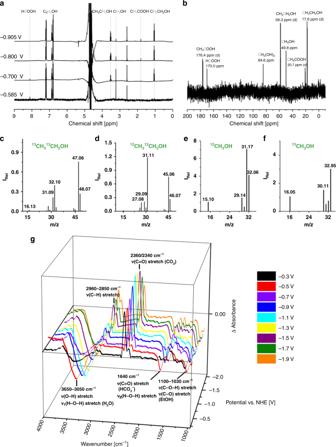Fig. 3 a1H-NMR spectrum of the electrolyte after 5 h of CO2electrolysis over Co-corrole–carbon paper electrode at −0.585, −0.7, −0.8, and −0.905 V vs. RHE in 0.1 M NaClO4, pH = 6, phosphate buffer, and phenol as the internal standard in DMSO.b13C-NMR (101 MHz, H2O:D2O = 5:1) of the electrolyte after 5 h of electrolysis at −0.8 V vs. RHE in13CO2, 0.1 M NaClO4, pH = 6, phosphate buffer.c–fGC–MS spectrum of the electrolyte after bulk electrolysis at −0.8 V vs. RHE in12CO2and13CO2:c13C enriched ethanol,d12C enriched ethanol,e12C enriched methanol, andf13C enriched methanol.gSEC-FTIR spectra during the CO2reduction with 20 mM Co-corrole in 0.1 M TBAPF6(in CH3CN/H2O = 4:1), at potentials from −0.3 to −1.9 V vs. NHE The catalyst physisorbed on carbon paper was subjected to X-ray photoelectron spectroscopy (XPS) analysis before (Supplementary Table 2 ) and after the electroreduction (Supplementary Table 3 ). XPS survey scans exhibited the corresponding Co2p, Co3p, N1s, F1s, S2s, S2p, and P2p binding energy regions (Supplementary Fig. 15 ). The observed peaks correspond to Co2p, F1s, and P2p in the spectrum of Co-corroles as well as the absence of these peaks in the spectrum of non-modified carbon paper confirmed the presence of Co-corrole on the carbon paper. The high-resolution Co2p and N1s XP spectra (Supplementary Fig. 15 ) are in good agreement with previously published XPS data from CoTPP multilayer films [41] , [51] . The main peak for Co 2p 3/2 at 780.18 eV, is located at a typical cobalt(II) position (e.g., 780.2 eV for CoO) and the main peak for N1s is at 398.53 eV. Supplementary Fig. 15 displays also a C1s XP spectrum taken after electrocatalysis reaction. We observe two signals at 284.6 and 286.2 eV, because not all aromatic carbon atoms in the Co-corrole are the same, due to a lowering of symmetry to C 2v for corroles relative to D 4h for porphyrins. The shake-up satellite at 289.0 eV is typical for organic molecules with extended conjugated π systems. The XPS scans show that the catalyst is stable in course of electrocatalysis (Supplementary Fig. 15 ). Heterogeneous CO 2 electroreduction The heterogeneous electrochemical CO 2 reduction experiments were carried out with Co-corrole deposited on carbon paper with effective loadings of 0.2 mg cm −2 . The modified electrode was found to reduce CO 2 to ethanol and methanol in 0.1 M NaClO 4 at a potential of −0.8 V vs. RHE (pH = 6.0, 0.1 M phosphate buffer, Table 1 ). Controlled potential electrolysis (CPE) under CO 2 of Co-corrole modified carbon paper exhibits a TON = 196 and a TOF = 0.011 s −1 for the catalytic conversion of CO 2 to EtOH over 5 h (Fig. 2a–d ). The quantification of products was performed using the observed 1 H-nuclear magnetic resonance (NMR)- and gas chromatography mass spectrometry (GC–MS) measurement (e.g., in Fig. 3a and Table 1 , and Supplementary Notes 1– 3 ). XPS analysis of the electrode materials before and after catalysis reveals that the catalyst is stable in course of electroreduction and the catalyst pertaining to the reduction process are molecular Co-corrole units (Supplementary Fig. 15 ). Moreover, in the course of 5 h electrolysis at −0.8 V vs. RHE the Faradaic efficiency (FE%) for the ethanol production was measured at different intervals of time (Fig. 2a ). Figure 2a illustrates that the FE = ~48% stays constant throughout the electrocatalytic reduction process. Subsequently, we have performed CPE with the modified carbon paper electrodes at different potentials, between −0.515 to −0.955 V vs. RHE for 5 h with current densities of 1.9–2.9 mA cm −2 . H 2 is the main gaseous compound and in the liquid phase ethanol, methanol, acetate, formaldehyde, glyoxal, and formate was detected. The quantifications of the respective gaseous and liquid compounds are summarized in Fig. 2b , c, Table 1 , and Supplementary Figs. 16 – 23 . During the CO 2 reduction process, the FE% for ethanol was found in the range of 9–48 with the selectivity for C 2 over C 1 increasing with increase in the applied cathodic potential from −0.73 to −0.96 V vs RHE with a significant decrease in methanol production. CPE long-term measurements were performed at −0.73 V (pH = 6.0) and −0.70 V (pH = 7.2) vs. RHE, where the activity of the Co-corrole modified carbon electrodes retained for 140 h (Supplementary Figs. 8 – 13 ). Table 1 Average Faradaic efficiency for each product detected on the Co-corrole-carbon paper electrode Full size table Fig. 2 a Constant potential electrolysis of electrochemical CO 2 reduction by the Co-corrole modified carbon paper electrode at a potential of −0.8 V vs. RHE (black curve), Faradaic efficiency for ethanol production over 5 h electrolysis (blue rectangles). b FE% vs. potential plot for potential dependent product formation. c FE% vs. potential plot for minor formed formaldehyde and solvated dimer of formaldehyde at different potentials. The error bars represent standard deviation of six measurements (three electrochemical reactions with two product analysis measurements for each reaction). d MS spectra obtained after electrolysis at −0.8 V vs. RHE in (1:3) D 2 O/H 2 O 0.1 M NaClO 4 saturated with CO 2 Full size image Fig. 3 a 1 H-NMR spectrum of the electrolyte after 5 h of CO 2 electrolysis over Co-corrole–carbon paper electrode at −0.585, −0.7, −0.8, and −0.905 V vs. RHE in 0.1 M NaClO 4 , pH = 6, phosphate buffer, and phenol as the internal standard in DMSO. b 13 C-NMR (101 MHz, H 2 O:D 2 O = 5:1) of the electrolyte after 5 h of electrolysis at −0.8 V vs. RHE in 13 CO 2 , 0.1 M NaClO 4 , pH = 6, phosphate buffer. c – f GC–MS spectrum of the electrolyte after bulk electrolysis at −0.8 V vs. RHE in 12 CO 2 and 13 CO 2 : c 13 C enriched ethanol, d 12 C enriched ethanol, e 12 C enriched methanol, and f 13 C enriched methanol. g SEC-FTIR spectra during the CO 2 reduction with 20 mM Co-corrole in 0.1 M TBAPF 6 (in CH 3 CN/H 2 O = 4:1), at potentials from −0.3 to −1.9 V vs. NHE Full size image To further trace the origin of methanol and ethanol, we carried out CO 2 reduction experiments with a D 2 O/H 2 O mixture. Deuterium distribution during the CO 2 reduction process was monitored by conducting electrolysis at −0.8 V vs. RHE in D 2 O/H 2 O (1:3). After electrolysis, the mass spectra indicated the formation of reduced product and the following peaks appeared— m / z of 45–52 (Fig. 2d ). Among the peaks obtained, the one with m / z value 52 (CD 3 CD 2 OD) can be assigned for hexa-deuterated ethanol. In the spectrum apart from the molecular ion peak, there are also peaks corresponding to other fragments with m / z = 50 which can be from CD 3 CD 2 O and m / z = 34 for CD 2 OD + which are characteristic fragments of CD 3 CD 2 OD . This deuteration further proves that the source and incorporation of protons in the reduced product is from the solvent and the source of ethanol is from CO 2 reduction. To confirm the source of carbon in the reduction products, we have conducted the reduction experiments with 12 CO 2 and 13 CO 2 . The 1 H and 13 C-NMR spectra after CO 2 reduction at the Co-corrole modified carbon paper electrode exhibit resonances for ethanol, methanol, acetic acid, and formic acid (Fig. 3a, b ). The 13 C-NMR spectrum after the reduction of 13 CO 2 clearly indicates four doublets at 58.3 ppm ( 1 J CC,EtOH = 37.5 Hz), 17.6 ppm ( 1 J CC,EtOH = 37.5 Hz), 176.4 ppm ( 1 J CC, acetic acid = 56.2 Hz), and 20.7 ppm ( 1 J CC, acetic acid = 56.2 Hz) indicating the reduction of 13 CO 2 and formation of C–C bond (Fig. 3b ). HCOOH and CH 3 OH appear as singlets at 170.0 and 49.8 ppm in the 13 C-NMR spectrum (Fig. 3b ), respectively. These results were further substantiated by GC–MS data, which shows a shift of m / z = 2 for the molecular ion peak of CH 3 CH 2 OH + on 13 C enrichment (Fig. 3c, d ). The results for CH 3 OH + , when compared to 12 CO 2 reduction shows a shift by m / z = 1 (Fig. 3e, f ). On analysis of the fragmentation patterns, we observe that for ethanol obtained by the reduction of 12 CO 2 , the peak at m / z = 29 corresponds to the CH 3 CH 2 + ion. On the other hand, when 13 CO 2 is used, the peak occurs at m / z = 31, which is due to the substitution of both 12 C centers with 13 C isotopes. Likewise, the peak obtained at m / z = 31 in case of 12 C enriched ethanol resembles the CH 2 OH + fragment which on 13 C enrichment shifts to m / z = 32. For 12 C enriched methanol, the peak at m / z = 15 resembles CH 3 + ion which shifts to m / z = 16 on 13 C enrichment. The results obtained from both the 13 C-NMR and GC–MS experiments prove that the source of ethanol as well as methanol is CO 2 (Fig. 3b–f ). Spectroelectrochemical Fourier-transform infrared spectroscopy (FTIR) measurements (SEC-FTIR) at applied potentials of −0.3 to −1.9 V vs. NHE, illustrated in Fig. 3g exhibit increasing IR bands at 3400 cm −1 (O–H stretching), 2960 cm −1 (C–H stretching), 2850 cm −1 (C–H stretching), 1100–1060 cm −1 (C–O stretching), indicating the stepwise increase of [alcohol/acid] formation. The IR-band at 1640 cm −1 (C = O stretching of HCO 3 − ) indicates the formation of a bicarbonate species. The corresponding IR bands for CO 2 at 2360 and 2340 cm −1 (C = O stretching CO 2 ) decrease during the reaction, indicating that CO 2 is converted under these conditions. An in-depth elucidation of the mechanistic pathway of the reduction process is beyond the scope of this present work. Detailed investigations are underway in our laboratories. To increase the CO 2 reduction efficiency and to avoid hydrogen evolution at low-pH values, all experiments were performed under weak acidic conditions (pH = 6.0, 0.1 M phosphate buffer). CO 2 reduction under heterogenized conditions with Co-corrole modified carbon electrodes exhibits a redox couple being [Co-corrole] 1− /[Co-corrole] 2− , which was found to be at −0.8 V vs. RHE. This markedly resembles the redox behavior of the Co-corrole molecule in the solution, so the redox properties are unperturbed upon heterogenization. We thus propose the molecular characteristics of the electrocatalyst to be persistent upon heterogenization. The EPR spectrum obtained after electrochemical reduction and subsequent dosage of CO 2 at room temperature exhibits a rhombic S = 1/2 signal at g = 2 with a weak 59 Co hyperfine splitting and indicates the formation of Co(III)–CO 2 •− species (Supplementary Fig. 24 ). The role of protons is extremely crucial in this work and sets this process apart from related CO 2 reduction processes. For instance, at pH = 6.0 the necessary protons are provided for the subsequent proton coupled electron transfer (PCET), due to this, reduction to methanol/ethanol takes place (Fig. 3a ). By performing the same experiment at pH = 7.2, we experimentally observe the reduction of CO 2 to a mixture of formaldehyde, ethanol, methanol, acetate, and formate (see assignment of NMR resonances in the supplementary Fig. 20 ), and at a pH = 8.0 we detect only CO as the main reduction product (Supplementary Fig. 25a–c and Supplementary Notes 4, 5 ). This implies that the rate of PCET drastically decreases at weakly to moderately basic pH values. For the successful chemical transformation of CO 2 to methanol and ethanol, this result is crucial in the present context. The existence of the Co(III)–CO 2 •− can only be justified through the presence of CO 2 •− formed at a very high potential of ca . −1.5 V vs. RHE [52] . But in our case, the reduction wave at ca . −0.8 V vs. RHE is responsible for the CO 2 reduction. This implies that the Co(I) in the center of the corrole complex enables the reduction of CO 2 to the CO 2 •− intermediate at a lower cost of energy. We suggest a mechanism similar to that proposed by Koper et al. [53] . which is illustrated in Fig. 4 . The reaction follows a low energy pathway where the carboxyhydroxyl intermediate gets simultaneously reduced by 1 e − , gets protonated to form a HCO 2 H intermediate and can be detected by 1 H-NMR spectroscopy (Fig. 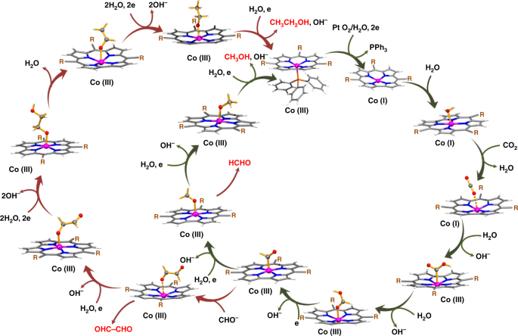Fig. 4 Proposed single site mechanism of CO2reduction using Co-corrole 3a , Supplementary Table 4 , and Supplementary Notes 6 – 8 ). The HCO 2 H intermediate further undergoes 1e − reduction with the elimination of OH − to give HCO • stabilized at the Co(III) site. Low potential for reactivity then drives the reaction toward methanol. This reduction pathway of HCO • to CH 3 O • at the cobalt site is in accordance with the mechanism reported by Koper et al. On the other hand, at a higher potential (>−0.73 V vs. RHE) an increased concentration of HCO • is developed and , the reaction takes a second route with the recombination of two formyl radicals (Co(III)–HCO • + HCO • ) leading to oxaldehyde intermediate (OHC–CHO). OHC–CHO was previously reported to be a precursor for the formation of ethanol as well as a key intermediate for C–C step-up leading to C 2 products [54] . The π-conjugation present in OHC–CHO inherently makes it prone to reduction giving • OCH 2 –CHO which subsequently reduces to • OCH 2 –CH 2 OH which further reduces to CH 3 CH 2 OH. The high selectivity for alcohol is due to the formation of the HCO • intermediate which is readily reducible to methanol. In the case of ethanol, we believe the formation of oxaldehyde intermediate opens up a more favorable route to form ethanol. Fig. 4 Proposed single site mechanism of CO 2 reduction using Co-corrole Full size image The proposed reaction pathways for the formation of the methanol and ethanol were further substantiated by conducting reduction studies of possible intermediates like formic acid, formaldehyde, methanol, and glyoxal under the same reaction conditions reported for Co-corrole–carbon paper electrodes. To test this conjecture, further reduction of the 2e − reduced product formic acid was induced, where it yielded a mixture of methanol and ethanol which indeed implies formic acid to be an important intermediate. Cyclic voltammetric measurements show an increase in current density (Supplementary Fig. 34a ) upon the addition of 10 mM of formic acid. CPE was performed at −0.73 V vs. RHE over Co-corrole–carbon paper for 5 h and the products obtained were analyzed in GC–MS spectrum where the presence of the characteristic peaks of methanol ( m / z = 32) and ethanol ( m / z = 46) were observed (Supplementary Figs. 36 – 38 ). The obtained results were further confirmed by 1 H-NMR spectroscopy (Supplementary Fig. 34b ). The proposed HCOOH intermediate under the low potential of reactivity gets reduced to HCHO and methanol, which are the final products and does not get further reduced. To verify the role of oxaldehyde in the current mechanistic cycle, 0.1 mM OHC–CHO was externally added under the reaction condition and CH 3 CH 2 OH was obtained proving oxaldehyde to be a key intermediate for CH 3 CH 2 OH formation (Supplementary Fig. 35a, b ). The high selectivity for alcohol is primarily due to the formation of the formic acid intermediate followed by formation of HCO • intermediate which is readily reducible to methanol. In the case of ethanol, we believe the formation of oxaldehyde is due to coupling of two HCO • intermediate which opens up a more favorable route to form ethanol. To complete the studies, we performed comparative measurements with two similar Co-corroles (cobalt triphenylphosphine 5,10,15–tris(pentafluoro-phenyl) corrole (PPh 3 -CoTpFPC) and cobalt triphenylphosphine 5,10,15–triphenyl corrole PPh 3 -CoTPC)), which consist of (a) three meso- C 6 F 5 -groups or of (b) three meso- C 6 H 5 -groups. The results are illustrated in the Supplmentary Informations file of the paper (Supplementary Fig. 43 ). The main reduction products under the same reaction conditions at pH = 6 were assigned to formic acid, methanol, and acetic acid. Only trace amounts of ethanol were found employing these two catalyst systems. To conclude, we have demonstrated the electrochemical reduction of CO 2 to ethanol and methanol with a Co-corrole–carbon paper electrode at a low potential (−0.8 V vs. RHE) with a FE of 48% over a time period of 5 h. The Co-corrole–carbon paper electrode can withstand extremely high operational time of up to 140 h marking the highest efficiency for a molecular electrocatalyst reported so far in the literature. This is accomplished by the formation of a OHC–CHO type intermediate using a MeO-PEG(7)-S-modified cobalt corrole molecular catalyst. The Co-corrole molecule tends to stabilize different radical intermediates at the metal site. Thus, when reacted with a greater number of electrons highly reduced products are formed. On simulating the reactivity of Co-corrole, we found both experimentally and theoretically that in contrast to the CO pathway our catalyst proceeds via a formic acid pathway. By applying a redox potential of −0.73 V vs. RHE, a mixture of methanol and ethanol is detected. The obtained reaction products can only be explained if formic acid is developed temporarily, which is subsequently reduced to the formyl radical (HCO • ). The HCO • forms methanol as well as glyoxal and ultimately the glyoxal is then reduced to form ethanol serving our catalyst to operate at a low over potential. Chemicals All chemicals and solvents were commercially available and were used as obtained, unless otherwise noted. High-performance liquid chromatography grade solvents were used in all the experiments with water, methanol, acetonitrile, and sodium perchlorate (NaClO 4 ) purchased from Merck, tetrabutylammonium perchlorate (Bu 4 NClO 4 ), and Ferrocene from Sigma Aldrich. Tetrabutylammonium hexafluorophosphate (Bu 4 NPF 6 ), 98%, purchased from Alfa Aesar, was twice recrystallized with absolute Ethanol, dried under high vacuum and stored under nitrogen. The 5,10,15-trispentafluorophenylcorrole was synthesized according to the Gryko’s method for highly reactive aldehydes [48] . For NMR experiments D 2 O was purchased from Cambridge Isotopic Laboratory. GC authentic standard ethanol, methanol, glyoxal, and diethoxymethane were purchased from Sigma Aldrich. Toray Carbon Paper, TGP-H-60, 19 × 19 cm was purchased from Alfa Aesar. 2,2,6,6-tetramethyl-1-piperidinyloxy, free radical, 2,2,6,6-tetramethylpiperidine 1-oxyl, TEMPO was purchased from Sigma Aldrich. 13 CO 2 (99.0 atom%) from Icon isotopes USA and Sigma Aldrich. CO 2 and Ar used in the electrochemical measurements were purchased from Praxair with a purity of 99.995%. Materials synthesis and characterization Free base 5,10,15-tris(2,3,5,6-tetrafluoro-4-(MeO-PEG(7))thiophenyl)corrole H 3 TpFPC(-S-PEG(7)-OMe) 3 250 mg 5,10,15-tris(pentafluorophenyl)corrole (H 3 TpFPC) (314 µmol) and 225 mg sodium hydride (60% in mineral oil, 30 equiv., 9.4 mmol) were given in a 250 mL two-neck round-bottom flask under argon atmosphere. Totally, 100 mL THF abs. and 336 mg MeO-PEG(7)-thiol (3 equiv., 942 µmol) were added and the reaction was stirred at room temperature for 30 min. The reaction was controlled via TLC and mass spectroscopy. To quench the reaction, 15 mL H 2 O dest. were added. Further saturated aqueous NH 4 Cl-solution was added and the solution was extracted three times with ethylacetate. The combined organic phases were washed with 0.1 M HCl, dried over Na 2 SO 4 , filtered and evaporated to dryness. The product H 3 TpFPC(-S-PEG(7)-OMe) 3 (517.8 mg, 0.267 mmol, 91.3 %) was obtained as a turquoise solid. 1 H-NMR (300.1 MHz, CDCl 3 , 25 °C): δ = 9.09 (2H, d, 3 J = 4.14 Hz, H2 + H18), 8.80 (2H, d, 3 J = 4.38 Hz, H7 + H13), 8.61–8.58 (4H, m, H8 + H12 + H3 + H17), 3.91 (6H, t, 3 J = 6.20 Hz, –CH 2 ), 3.74–3.71 (12H, m, –CH 2 ), 3.68–3.65 (12H, m, –CH 2 ), 3.61 (12H, bs, –CH 2 ), 3.56–3.55 (18H, m, –CH 2 ), 3.52–3.49 (6H, m, –CH 2 ), 3.42–3.39 (12H, m, –CH 2 ), 3.26 (9H, s, –CH 3 ) ppm (Supplementary Fig. 1 ). 19 F-NMR (282.4 MHz, CDCl 3 , 25 °C): δ = −133.63 (4F, dd, 3 J = 25.20 Hz, 4 J = 11.87 Hz, Fo), −134.06 (2F, dd, 3 J = 25.76 Hz, 4 J = 12.12 Hz, Fo), −137.56 (2F, dd, 3 J = 25.50 Hz, 4 J = 12.21 Hz, Fm), −138.22 (4F, dd, 3 J = 24.94 Hz, 4 J = 11.73 Hz, Fm) ppm (Supplementary Fig. 2 ). HRMS (ESI, positive): m / z calculated for C 82 H 104 F 12 N 4 O 21 S 3 : 1805.6236 [M+H] + , 1827.6061 [M + Na] + ; found: 1805.6273 [M + H] + , 1827.6096 [M + Na] + (Supplementary Fig. 3 ). Co-Corrole: Co(PPh 3 ) (TpFPC)(-S-PEG(7)-OMe) 3 Totally, 385.2 mg of H 3 TpFPC(-S-PEG(7)-OMe) 3 (0.213 mmol) were dissolved in 250 mL DCM: MeOH (2:1) in a 250 mL two-neck round-bottom flask under argon atmosphere. Cobalt(II)acetatetetrahydrate (539.7 mg, 2167 mmol, 10 equiv.) and triphenylphosphine (58.5 mg, 0.233 mmol, 1 equiv.) were added and the reaction mixture was heated to reflux for an hour. The reaction progress was monitored via UV/vis and TLC. After complete metalation, the mixture was extracted with DCM. The combined organic phases were extracted four times with water, dried over Na 2 SO 4 , filtered and evaporated under reduced pressure. Purification was performed with silica gel column chromatography (DCM/MeOH = 20:1), where the red product Co(PPh 3 )(TpFPC)(-S-PEG(7)-OMe) 3 was obtained with 54.4% yield (246.3 mg, 115.9 µmol). 1 H-NMR (300.1 MHz, CDCl 3 , 25 °C): δ = 8.68 (2H, d, 3 J = 4.50 Hz, H2 + H18), 8.36 (2H, d, 3 J = 4.77 Hz, H7 + H13), 8.26 (2H, d, 3 J = 4.74 Hz, H8 + H12) 8.12 (2H, d, 3 J = 4.47 Hz, H3 + H17), 7.04–6.99 (3H, m, triphenylphospine-CH), 6.69–6.64 (6H, m, triphenylphospine-CH), 4.64–4.58 (6H, m, triphenylphospine-CH), 3.91–3.86 (6H, m, –CH 2 ), 3.74–3.69 (24 H, m, –CH 2 ), 3.65–3.59 (42H, m, –CH 2 ), 3.52–3.49 (6H, m, –CH 2 ), 3.35 (9H, s, –CH 3 ) ppm (Supplementary Fig. 4 ). 19 F-NMR (282.4 MHz, CDCl 3 , 25 °C): δ = −133.88 to −133.72 (3F, m, Fo), −134.47 to −134.21 (3F, m, Fo), −136.99 (3F, dd, 3 J = 25.47 Hz, 4 J = 12.00 Hz, Fm), −137.30 (1F, dd, 3 J = 25.44 Hz, 4 J = 12.10 Hz, Fm), −138.08 (3F, dd, 3 J = 25.81 Hz, 4 J = 11.94 Hz, Fm) −138.44 (1F, dd, 3 J = 25.80 Hz, 4 J = 12.09 Hz, Fm) ppm (Supplementary Fig. 5 ). HRMS (APPI, positive): m / z calculated for C 82 H 104 F 12 N 4 O 21 S 3 : 2145.6064 [M + Na] + ; found: 2145.6078 [M + Na] + (Supplementary Fig. 6 ). Preparation of the working electrode The working electrode consists of cobalt(III)-corrole immobilized over carbon fiber paper ( A = 1 cm 2 ). For this, a 0.5 mmol solution of cobalt(III)-corrole in acetonitrile was prepared and drop-casted over carbon fiber to make a loading of 0.2 mg cm −2 . Further, we preserve the electrodes at room temperature to remove the excess acetonitrile. Then these electrodes were washed with 0.1 M pH = 6 phosphate buffer to get rid of the acetonitrile completely. Then the electrodes were dried in presence of CaCl 2 under high vacuum. Cyclic voltammetry and CPE Cyclic Voltammetry and CPE for CO 2 reduction were performed with a workstation (CH Instruments, Model CHI400A) in a two-compartment, three-electrode electrochemical H-cell, consisting of a gas tight cell with a total volume of 30 mL. Carbon paper was used as the working electrode. Ag/AgCl ( E Ag/AgCl = 0.222 V filled with 0.1 M KCl) as the reference, and Pt wire as the counter. The reference electrode potential was calibrated with respect to the reversible hydrogen potential using platinum working electrode and platinum wire as counter electrode in 0.5 M H 2 SO 4 electrolyte in H 2 atmosphere. This calibration result showed a shift of −0.222 V versus the NHE. All experiments were carried out at 25 °C. The pH value of the solutions were obtained using a EUTECH pH 510 pre-calibrated with Thermo Scientific pH 4.01, 7.0, and 10.01 buffer solutions. For all the measurements CO 2 was continuously purged into the solution. All the potentials are represented in RHE scale with iR correction. For electrochemistry in non-aqueous medium, acetonitrile was used as the solvent of choice with a similar electrochemical setup with glassy carbon as the working electrode, Ag/AgCl (0.1 M KCl) as the reference and Pt wire as the counter electrode with 0.1 M tetrabutylammonium perchlorate or 0.1 M tetrabutylammonium hexafluorophosphate as the electrolyte. Under this electrochemical conditions, the redox behavior of 0.01 M ferrocene in acetonitrile was studied, which was further used as the internal standard. Detection and quantification of the CO 2 reduced products 1 H- and 13 C-NMR spectroscopy of the carbon dioxide reduced liquid products were recorded a on a Bruker Ascend 700 MHz Avance III NMR spectrometer equipped with a cryoprobe and on a JEOL ECS-400 NMR spectrometer. As internal standard, 20 mL aqueous solution of 20 mM phenol and 10 mM of dimethyl sulfoxide were used. After CPE, to 350 µL electrolyte, 200 µL D 2 O, and 50 µL of the internal standard were added and transferred into a NMR-tube. During the measurements, the water peak was suppressed to increase the signal intensity of the analytes. The CO 2 reduced products were further analyzed using GC–MS. Trace 1300 GC and ISQ QD single quadruple GC–MS instrument with a TG-5MS capillary column (30 m × 0.32 mm × 0.25 µm) supplied by Thermo Fisher Scientific and DB-624 capillary column (30 m × 0.32 mm × 0.25 µm) supplied by Agilent were used for the same. For gaseous analysis CarboPLOT 007 capillary column (25 m × 0.53 mm × 0.25 µm) supplied by Agilent was used for separation and TCD for detection. Electrochemically active surface area (ECSA) calculation ECSA value is obtained by using the following equation 
    ECSA = C_D/C_S
 (1) where C D = electrochemical double layer capacitance which is obtained from the slope of the current vs. scan rate plot in the non-Faradaic region and C S = specific capacitance of the sample and in this case, C S = 0.040 mF cm −2 [55] . Analysis of the CO 2 reduced products in 1 H-NMR and GC–MS Compounds formed at different potentials were detected directly by 1 H-NMR (integrated with respect to DMSO ( δ = 2.71 ppm) as an internal standard) with a triplet signal at δ = 1.17 ppm and a quartet at δ = 3.67 ppm indicating ethanol (Supplementary Fig. 17 ); a singlet at δ = 3.37 ppm showing the presence of methanol (Supplementary Fig. 17 ). For detection of formaldehyde, 2 mL of the reaction mixture was taken in a 20 ml headspace vial with 25 μL of ethanol and was acidified with 100 μL 1% p -toluenesulfonic acid. This mixture was then heated at 60 °C for 1 h and then GC–MS measurements were done [56] . In the mass spectrum, peak centered at m / z = 104 represents diethoxymethane indicating the formation of formaldehyde with a retention time around 3.00 min (Supplementary Figs. 39 and 40 ). Glyoxal was detected in the spectrum at m / z = 58 with a retention time of 3.35 min (Supplementary Figs. 41 and 42 ). XPS measurements XPS was performed by using a Theta Probe, Thermofisher, UK, using monochromatic Al Kα X-rays ( hν = 1486.6 eV), spot size 400 microns and with a photoelectron take-off angle of 90° with respect to the surface plane. The binding energies were corrected using the C1s peak at BE = 284.6 eV that arises from adventitious hydrocarbon.